Identification of renin progenitors in the mouse bone marrow that give rise to B-cell leukaemia The cell of origin and triggering events for leukaemia are mostly unknown. Here we show that the bone marrow contains a progenitor that expresses renin throughout development and possesses a B-lymphocyte pedigree. This cell requires RBP-J to differentiate. Deletion of RBP-J in these renin-expressing progenitors enriches the precursor B-cell gene programme and constrains lymphocyte differentiation, facilitated by H3K4me3 activating marks in genes that control the pre-B stage. Mutant cells undergo neoplastic transformation, and mice develop a highly penetrant B-cell leukaemia with multi-organ infiltration and early death. These renin-expressing cells appear uniquely vulnerable as other conditional models of RBP-J deletion do not result in leukaemia. The discovery of these unique renin progenitors in the bone marrow and the model of leukaemia described herein may enhance our understanding of normal and neoplastic haematopoiesis. Renin cells have traditionally been associated with the regulation of blood pressure and fluid-electrolyte homeostasis. Pursuing the mechanisms that regulate the identity of these cells, we uncovered an unexpected property of renin cells in the bone marrow with relevance to the development of malignancy. Renin progenitors appear early in the embryo and give rise to many different cell types throughout the body [1] . Whereas the function of renin cells in extra renal tissues is unclear, the ontogeny and function of renin cells in the kidney are better understood [2] , [3] , [4] , [5] . In the embryonic kidney, renin precursors are distributed extensively along nephrovascular units and participate in the assembly and branching morphogenesis of the kidney arterioles. As development of the kidney proceeds, renin precursors differentiate in situ into arteriolar smooth muscle cells, glomerular mesangial cells and interstitial pericytes. Thus, in the adult only a few cells at the tip of the renal arterioles near the glomeruli, the juxtaglomerular (JG) cells, retain the ability to synthesize and secrete renin upon physiological demands [1] . Under normal conditions, those cells suffice to regulate blood pressure and fluid-electrolyte homeostasis. However, if such adult animal is subjected to a homeostatic threat (such as hypotension, dehydration, sodium depletion or administration of renin–angiotensin inhibitors), there is an increase in the number of renin-expressing cells along the arterioles, glomeruli and interstitium, resembling the embryonic pattern described above [6] , [7] . This phylogenetically conserved process occurs by re-transformation of arteriolar smooth muscle cells, mesangial cells and pericytes into renin-expressing cells [1] , [8] . Because renin cells contain all the components of the Notch pathway including RBP-J, the final transcriptional effector of all the Notch receptors [9] , and Notch/RBP-J is known to regulate cell fate, we previously examined whether deletion of RBP-J regulates the identity and plasticity of kidney renin cells during normal development and in response to a physiological threat. Conditional deletion of RBP-J in renin-expressing cells resulted in a decrease in the number of renin-positive JG cells in the kidney and an inability of smooth muscle cells along the kidney vasculature to regain the renin phenotype [10] . Unexpectedly, as these mice aged beyond 6 months, they developed signs and symptoms of a highly penetrant and fulminant form of precursor B-lymphoblastic leukaemia. Given the potential medical relevance of this finding, in this study we perform an extensive series of experiments to fully characterize this mouse model of leukaemia, including its natural history and the genomic and epigenetic events underlying its development. We also set out to identify, and characterize in detail, which cells in the bone marrow are capable of producing renin under normal circumstances and whether those cells may be the origin of this striking model of leukaemia. Finally, we ascertain whether mutations in the RBP-J gene are associated with leukaemia in humans as well. We find that renin is expressed by a subset of B-cell progenitors in the mouse bone marrow, and that these renin-expressing cells are the cell of origin for B-cell leukaemia when RBP-J is deleted. Deletion of RBP-J in renin cells results in B-cell leukaemia We deleted RBP-J in cells of the renin-lineage by crossing mice that express Cre recombinase under control of the renin locus with RBP-J fl/fl mice [1] , [10] , [11] . Mutant mice ( RBP-J fl/fl ; Ren1 dcre/+ ) developed progressive abdominal distension and poor overall health by ~6 months of age ( Fig. 1a ). Necropsy demonstrated massive hepatosplenomegaly (spleen and liver weights were 15- and 4-fold higher than controls, respectively) ( Fig. 1a–d ). Mutant animals displayed marked leukocytosis and anaemia ( Fig. 1e ), lymph node tumour formation (74% of mutant mice developed axillary or retroperitoneal tumours) ( Fig. 1f ), and succumbed at an early age with a median survival of 269 days ( Fig. 1g ). 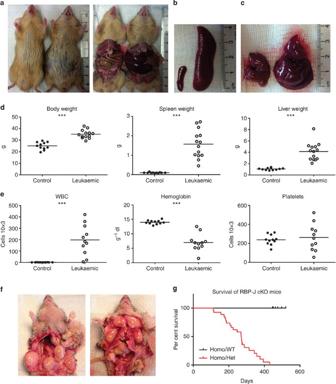Figure 1: Deletion ofRBP-Jin renin-lineage cells leads to tumour development and early death. (a) Mutant mice (right in both panels) develop abdominal distension compared with control mice (left in both panels) and necropsy demonstrated that abdominal distension was due to hepatosplenomegaly. (b) Representative picture of enlarged spleen from mutant mouse (right) compared with control (left). (c) Representative picture of the enlarged liver from mutant mouse (right) compared with control (left). (d) Leukaemic mice have statistically significant increased body, spleen and liver weights compared with control mice. Student’st-test; ***P<0.001 (n=11 for control mice andn=14 for mutant mice). (e) The white blood cell (WBC) count is significantly higher and haemoglobin lower in leukaemic mice compared with controls. The platelet count is not significantly different between control and leukaemic mice. Horizontal lines represent the mean for each group in panels d-e. Student’st-test; ***P<0.001 (n=11 for both control mice and mutant mice). (f) Lymphomatous tumours (yellow asterisks) at lower extremities, abdomen, anterior neck and upper extremities. Tumours were commonly found in the retroperitoneum just anterior to the vertebral column. (g) Kaplan–Meier survival curve showing early death of leukaemic mice compared with control mice. Figure 1: Deletion of RBP-J in renin-lineage cells leads to tumour development and early death. ( a ) Mutant mice (right in both panels) develop abdominal distension compared with control mice (left in both panels) and necropsy demonstrated that abdominal distension was due to hepatosplenomegaly. ( b ) Representative picture of enlarged spleen from mutant mouse (right) compared with control (left). ( c ) Representative picture of the enlarged liver from mutant mouse (right) compared with control (left). ( d ) Leukaemic mice have statistically significant increased body, spleen and liver weights compared with control mice. Student’s t -test; *** P <0.001 ( n =11 for control mice and n =14 for mutant mice). ( e ) The white blood cell (WBC) count is significantly higher and haemoglobin lower in leukaemic mice compared with controls. The platelet count is not significantly different between control and leukaemic mice. Horizontal lines represent the mean for each group in panels d-e. Student’s t -test; *** P <0.001 ( n =11 for both control mice and mutant mice). ( f ) Lymphomatous tumours (yellow asterisks) at lower extremities, abdomen, anterior neck and upper extremities. Tumours were commonly found in the retroperitoneum just anterior to the vertebral column. ( g ) Kaplan–Meier survival curve showing early death of leukaemic mice compared with control mice. Full size image Blood smears from mutant mice demonstrated a predominance of lymphoblasts ( Fig. 2a ). Flow cytometry of bone marrow and tumours confirmed the presence of an aberrant B-lymphoid (B220 dim /CD19 + ) immunophenotype at the expense of myeloid cells compared with control mice ( Fig. 2b ). The phenotype was indicative of precursor B-cell leukaemia evidenced by the lack of IgM and IgD expressions ( Fig. 2c ). Similar findings were found in the spleen and peripheral blood of leukaemic animals ( Supplementary Fig. 1a–c ). 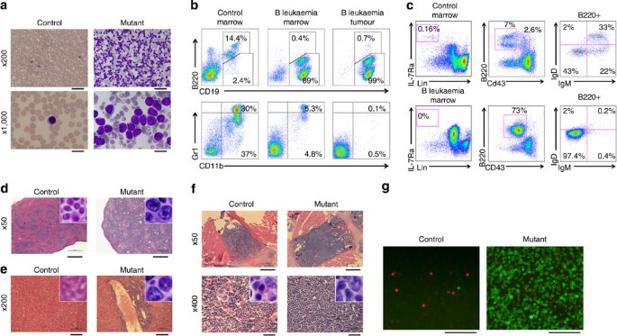Figure 2: Deletion ofRBP-Jin renin-lineage cells results in cell autonomous precursor B-cell leukaemia with infiltration of multiple organs. (a) May–Grunwald Giemsa-stained blood smears from control and mutant mice at low and high power. Scale bars equal 100 μm (top row) and 20 μm (bottom row). (b) Representative flow cytometric analysis of bone marrow. Control mice (left column) show 14.4% B cells with normal immunophenotype (B220+CD19+, top), 30% granulocytes (Gr1+CD11b+, bottom) and 37% immature myeloid cells (GR1−CD11b+). Leukaemic mice (middle column) show a significant reduction in normal B cells (0.4%), granulocytes (5.3%) and immature myeloid cells (4.8%), and a markedly expanded population of lymphoblasts (89%) with aberrant dim B220 expression (B220DimCD19+). (c) Representative flow cytometric analysis of bone marrow from control and leukaemic mice demonstrating arrest of B-cell maturation. Control marrow contains 0.16% of common lymphocyte progenitors (Lin−IL7Rα+) compared with ~0% in leukaemic marrow (left column). Control marrow contains 2.6% of pro B cells (B220+CD43+) and 7% of B220+CD43−B cells (middle), that correspond 43% to pre B cells (B220+CD43−IgM−IgD−), 22% to immature B cells (B220+CD43−IgM+IgD−) and 33% to mature B cells (B220+CD43−IgM+IgD+) (right). The leukaemic marrow has a large population of B220+CD43+cells (73%) (middle) similar to a pro B-cell population, and minimal IgM or IgD expression marking the lymphoblasts as precursor B-cell leukaemia (right). (d) Haematoxylin and eosin staining of spleen sections from control and mutant mice. Scale bar, 500 μm. (e) Haematoxylin and eosin staining of liver sections from control and mutant mice. Scale bar, 100 μm. (f) Low and high magnification of bone marrow. Scale bar, 500 μm (top row) and 50 μm (bottom row). Insets show higher magnification of lymphoid cells (d–f). (g) Fluorescence of peripheral blood from control and mutant mice withmT/mGreporter demonstrates expansion of the GFP+-cell population in mutant mice. Scale bar, 100 μm. Figure 2: Deletion of RBP-J in renin-lineage cells results in cell autonomous precursor B-cell leukaemia with infiltration of multiple organs. ( a ) May–Grunwald Giemsa-stained blood smears from control and mutant mice at low and high power. Scale bars equal 100 μm (top row) and 20 μm (bottom row). ( b ) Representative flow cytometric analysis of bone marrow. Control mice (left column) show 14.4% B cells with normal immunophenotype (B220 + CD19 + , top), 30% granulocytes (Gr1 + CD11b + , bottom) and 37% immature myeloid cells (GR1 − CD11b + ). Leukaemic mice (middle column) show a significant reduction in normal B cells (0.4%), granulocytes (5.3%) and immature myeloid cells (4.8%), and a markedly expanded population of lymphoblasts (89%) with aberrant dim B220 expression (B220 Dim CD19 + ). ( c ) Representative flow cytometric analysis of bone marrow from control and leukaemic mice demonstrating arrest of B-cell maturation. Control marrow contains 0.16% of common lymphocyte progenitors (Lin − IL7Rα + ) compared with ~0% in leukaemic marrow (left column). Control marrow contains 2.6% of pro B cells (B220 + CD43 + ) and 7% of B220 + CD43 − B cells (middle), that correspond 43% to pre B cells (B220 + CD43 − IgM − IgD − ), 22% to immature B cells (B220 + CD43 − IgM + IgD − ) and 33% to mature B cells (B220 + CD43 − IgM + IgD + ) (right). The leukaemic marrow has a large population of B220 + CD43 + cells (73%) (middle) similar to a pro B-cell population, and minimal IgM or IgD expression marking the lymphoblasts as precursor B-cell leukaemia (right). ( d ) Haematoxylin and eosin staining of spleen sections from control and mutant mice. Scale bar, 500 μm. ( e ) Haematoxylin and eosin staining of liver sections from control and mutant mice. Scale bar, 100 μm. ( f ) Low and high magnification of bone marrow. Scale bar, 500 μm (top row) and 50 μm (bottom row). Insets show higher magnification of lymphoid cells ( d – f ). ( g ) Fluorescence of peripheral blood from control and mutant mice with mT/mG reporter demonstrates expansion of the GFP + -cell population in mutant mice. Scale bar, 100 μm. Full size image Given the presence of lymphoblasts within the blood and bone marrow and the extensive organomegaly, we performed a comprehensive histologic evaluation of mutant and control mice. The spleens of mutant mice were massively infiltrated with lymphoblasts resulting in defacement of their normal architecture without recognizable red or white pulp ( Fig. 2d ). Lymphoblasts invaded the liver in a periportal and perisinusoidal distribution ( Fig. 2e ) and kidney interstitium ( Supplementary Fig. 2a ). Mutant mice developed skin lesions (characterized by loss of fur, nodules and ulcerations due to epidermal and dermal lymphoblastic infiltration) and lymphoid tumours ( Supplementary Fig. 2b,c ). Finally, bone marrow from leukaemic animals was hypercellular compared with controls and consisted of a homogenous blast population that occupied over 90% of marrow space ( Fig. 2f ). These blasts replaced other haematopoietic cells explaining the marked anaemia found in mutant animals. Lymphoblasts displayed diffuse and strong immunoreactivity for PAX5 and CD79a, further confirming a B-cell lineage and expressed TdT and CD34 supporting a B-cell precursor maturational stage ( Supplementary Fig. 2d–g ). To follow the distribution of mutant cells, we bred our mutant and control mice with mT/mG reporter mice, which normally express RFP in all cells but GFP only in cells that express Cre recombinase . Therefore, cells harbouring the RBP-J deletion are GFP + , whereas non-mutant leukocytes are RFP + [12] . The number of GFP + cells was markedly elevated in the blood and organs of mutant mice ( Fig. 2g ), indicating that deletion of RBP-J causes B-cell leukaemia with expansion of lymphoblasts to the bloodstream and invasion and morphological distortion of peripheral organs. Following the current classification of murine lymphoid neoplasms, the majority (92%) of mutant mice ( n =22) developed precursor B-cell lymphoblastic lymphoma/leukaemia (pre-B LBL) [13] . A minority (8%) of mice ( n =2) was affected by a myeloproliferative or mixed lymphoid/myeloid disorder and three animals developed mild disease. Given the striking predominance of the pre-B LBL, we focused our efforts on a detailed characterization of this phenotype. We performed multiple experiments to investigate if this leukaemia model represents a clonal process and if the leukaemic cells can grow in a cell-autonomous manner in culture and transplant systems. First, analysis of immunoglobulin gene rearrangements was performed to determine the clonal nature of leukaemic cells. These studies demonstrated that B cells from the spleen and bone marrow of mutant animals had unique patterns of V(D)J H rearrangements when compared with wild-type animals, with a predominant recombination indicating mono- or oligo-clonal IgH patterns ( Supplementary Fig. 3a–c ). Next, we performed colony-forming assays from bone marrow cells of mutant mice to determine the clonogenic potential of leukaemic cells. Whereas wild-type bone marrow did not form colonies beyond the first passage, leukaemic cells continue to grow even after extensive passaging. At the time of writing this manuscript, the leukaemic cell lines continue to be passaged, with one line currently beyond 25 passages, over 6 months ( Fig. 3a,b ). This cell line that expresses GFP (we bred mutant mice with mT/mG reporter mice) was chosen for extended analysis in transplant and gene expression studies. Deletion of RBP-J in this cell line was confirmed by PCR. To test whether those leukaemic cells are transplantable, GFP + cells from the aforementioned colonies were injected into the tail vein of irradiated host animals. At 1 week post injection, recipient animals were killed and organs were collected. While irradiated recipients that did not receive leukaemic cell injections had severely hypoplastic bone marrow, animals that received injections of leukaemic cells had a nearly normocellular marrow almost entirely composed of transplanted GFP + leukaemic cells ( Fig. 3c ). Further, leukaemic cells infiltrated multiple other organs including the spleen, lung, kidney, thymus and gonads as determined by the presence of massive numbers of GFP + cells ( Supplementary Fig. 4 ). Finally, GFP + leukaemic cells from the bone marrow of transplanted recipient animals were recovered and placed back into culture. The cells continue to grow in methycellulose, currently at passage 6, demonstrating the aggressive and resilient nature of these cells ( Fig. 3a ). Together, these studies indicate that deletion of RBP-J in renin cells results in leukaemic transformation as evidenced by clinical assessment, histologic evaluation, flow cytometry analysis, immunoglobulin rearrangements, colony-forming assays and transplantation studies. 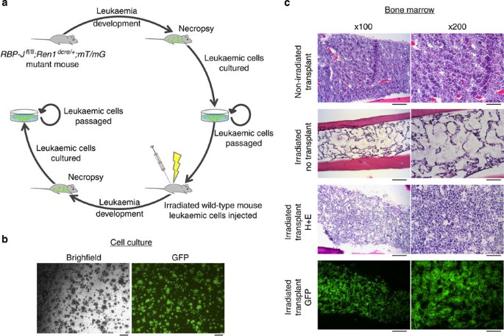Figure 3: Leukaemic cells grow in culture and are transplantable into irradiated mice. (a) Mutant animals expressing GFP (RBP-Jfl/fl;Ren1dcre/+;mTmG) developed leukaemia as described. When animals became moribund, necropsy was performed and bone marrow cells were collected for culture in methylcellulose. Cultured leukaemic cells are GFP+, have deletion ofRBP-J, have gene expression patterns similar to leukaemic spleens and can be serially passaged over many months. Leukaemic cells from culture were then injected into irradiated wild-type mice with engraftment and infiltration of GFP+-leukaemic cells. Bone marrow cells were recovered from transplanted animals and continued to grow in methylcellulose culture. (b) Leukaemic cells grow as colonies in methylcellulose culture. The population of leukaemic cells is homogenous. Scale bar, 200 μm. (c) In non-irradiated mice, leukaemic cells failed to engraft following intravenous injection. These animals had normocellular bone marrow (top row) and almost no presence of GFP+cells (0 to 4 GFP+cells per bone marrow section). Irradiated animals that received only injection of vehicle control (media) had markedly hypocellular bone marrow (second row) and absence of GFP+cells. Animals that received irradiation and injection of leukaemic cells had a mildly hypocellular bone marrow (third row) with almost all of the marrow cells expressing GFP (bottom row) demonstrating engraftment of leukaemic cells (n=3). Scale bar, 200 μm (left column) and 100 μm (right column). Figure 3: Leukaemic cells grow in culture and are transplantable into irradiated mice. ( a ) Mutant animals expressing GFP ( RBP-J fl/fl ;Ren1 dcre/+ ;mTmG ) developed leukaemia as described. When animals became moribund, necropsy was performed and bone marrow cells were collected for culture in methylcellulose. Cultured leukaemic cells are GFP + , have deletion of RBP-J , have gene expression patterns similar to leukaemic spleens and can be serially passaged over many months. Leukaemic cells from culture were then injected into irradiated wild-type mice with engraftment and infiltration of GFP + -leukaemic cells. Bone marrow cells were recovered from transplanted animals and continued to grow in methylcellulose culture. ( b ) Leukaemic cells grow as colonies in methylcellulose culture. The population of leukaemic cells is homogenous. Scale bar, 200 μm. ( c ) In non-irradiated mice, leukaemic cells failed to engraft following intravenous injection. These animals had normocellular bone marrow (top row) and almost no presence of GFP + cells (0 to 4 GFP + cells per bone marrow section). Irradiated animals that received only injection of vehicle control (media) had markedly hypocellular bone marrow (second row) and absence of GFP + cells. Animals that received irradiation and injection of leukaemic cells had a mildly hypocellular bone marrow (third row) with almost all of the marrow cells expressing GFP (bottom row) demonstrating engraftment of leukaemic cells ( n =3). Scale bar, 200 μm (left column) and 100 μm (right column). Full size image Renin cells in haematopoietic organs are precursor B cells To investigate the cell of origin and identity of the renin-expressing cell in the bone marrow and spleen, we used several strategies. First, we employed lineage tracing: we crossed Ren1 dcre/+ mice with mT/mG reporter mice that after Cre -mediated recombination express GFP in cells that expressed renin [12] . Fluorescence imaging demonstrated GFP + cells from the renin lineage in the spleen ( Fig. 4a ) and bone marrow ( Fig. 4b ), confirming the presence of cells from the renin lineage within these haematopoietic organs. RT–PCR confirmed the presence of renin mRNA in the bone marrow from control mice ( Supplementary Fig. 5a ). 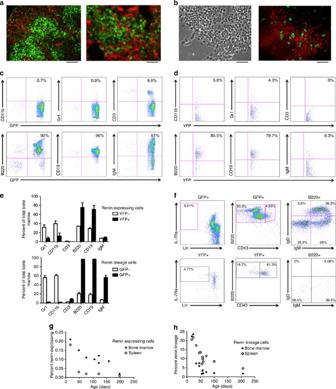Figure 4: Renin cells represent a small and diminishing population of B lymphocytes. (a) Low (left) and high (right) magnification fluorescence images of spleens fromRen1dcre/+;mT/mGmice. Scale bar, 100 μm (left) and 50 μm (right). (b) Bright-field (left) and fluorescence (right) images of the bone marrow fromRen1dcre/+;mT/mGmice showing the presence of GFP+renin-lineage cells. Scale bar, 50 μm. (c) Representative flow cytometry on the bone marrow fromRen1dcre/+;mT/mGmice demonstrating that renin-lineage cells (GFP+) express cell surface antigens most consistent with B cells (92% B220+, 96% CD19+and 61% IgM+) with minimal staining for markers of myeloid (<1% CD11b+and Gr1+) and T (<10% CD3+) cells. (d) Representative flow cytometry on bone marrow fromRen1c-YFPtransgenic mice demonstrating that renin-expressing cells (YFP+) are precursor B cells (85.5% B220+, 79.7% CD19+) with minimal staining for markers of more mature B cells (8.3% IgM+), myeloid cells (5.8% CD11b+and 4.3% Gr1+) and T cells (0% CD3+). (e) A comparison of YFP−versus YFP+(top) and GFP−versus GFP+(bottom) cell immunophenotypes in the bone marrow ofRen1c-YFPandRen1dcre/+;mT/mGreporter mice. Error bars represent s.e.m. (n=2 for renin-expressing (Ren1c-YFP) experiments andn=4 for renin-lineage (Ren1dcre/+;mT/mG) experiments). (f) Top panel: renin-lineage cells from the bone marrow were evaluated for cell surface markers consistent with common lymphocyte progenitors (Lin−IL-7Ra+), pro-B cells (B220+CD43+), premature B cells (B220+CD43−IgM−IgD−), immature B cells (B220+CD43−IgM+IgD−) and mature B cells (B220+CD43−IgM+IgD+). This strategy demonstrated that renin-lineage cells are ~0.01% common lymphocyte progenitors, <5% pro-B cells, ~33% premature B cells, ~24% immature B cells, and ~34% mature B cells. Bottom panel: renin-expressing cells were evaluated using the same strategy. This demonstrated that renin-expressing cells are predominantly (81.3%) pro-B cells with smaller populations of common lymphocyte progenitors (4.77%), pre-B cells (10.9%), immature B cells (6.8%) and mature B cells (0.95%). Images are representative of experiments performed in triplicate. (g) The percentage of renin-expressing (YFP+) cells within the bone marrow and spleen was quantitated over time usingRen1c-YFPmice and flow cytometry. Shortly, after birth, mice had ~0.2% renin-expressing cells. However, this percentage decreased with age in both the spleen and marrow to ~0.01%.n=8 for bone marrow samples andn=5 for spleen samples. (h) The percentage of renin-lineage (GFP+) cells within the bone marrow and spleen ofRen1dcre/+;mT/mGmice as measured by flow cytometry. The percentage of renin-lineage cells decreases from ~20% shortly after birth to ~2% at 200 days of life in the bone marrow.n=12 for both bone marrow and spleen samples. Figure 4: Renin cells represent a small and diminishing population of B lymphocytes. ( a ) Low (left) and high (right) magnification fluorescence images of spleens from Ren1 dcre/+ ;mT/mG mice. Scale bar, 100 μm (left) and 50 μm (right). ( b ) Bright-field (left) and fluorescence (right) images of the bone marrow from Ren1 dcre/+ ;mT/mG mice showing the presence of GFP + renin-lineage cells. Scale bar, 50 μm. ( c ) Representative flow cytometry on the bone marrow from Ren1 dcre/+ ;mT/mG mice demonstrating that renin-lineage cells (GFP + ) express cell surface antigens most consistent with B cells (92% B220 + , 96% CD19 + and 61% IgM + ) with minimal staining for markers of myeloid (<1% CD11b + and Gr1 + ) and T (<10% CD3 + ) cells. ( d ) Representative flow cytometry on bone marrow from Ren1 c -YFP transgenic mice demonstrating that renin-expressing cells (YFP + ) are precursor B cells (85.5% B220 + , 79.7% CD19 + ) with minimal staining for markers of more mature B cells (8.3% IgM + ), myeloid cells (5.8% CD11b + and 4.3% Gr1 + ) and T cells (0% CD3 + ). ( e ) A comparison of YFP − versus YFP + (top) and GFP − versus GFP + (bottom) cell immunophenotypes in the bone marrow of Ren1 c -YFP and Ren1 dcre/+ ;mT/mG reporter mice. Error bars represent s.e.m. ( n =2 for renin-expressing ( Ren1 c -YFP ) experiments and n =4 for renin-lineage ( Ren1 dcre/+ ;mT/mG ) experiments). ( f ) Top panel: renin-lineage cells from the bone marrow were evaluated for cell surface markers consistent with common lymphocyte progenitors (Lin − IL-7Ra + ), pro-B cells (B220 + CD43 + ), premature B cells (B220 + CD43 − IgM − IgD − ), immature B cells (B220 + CD43 − IgM + IgD − ) and mature B cells (B220 + CD43 − IgM + IgD + ). This strategy demonstrated that renin-lineage cells are ~0.01% common lymphocyte progenitors, <5% pro-B cells, ~33% premature B cells, ~24% immature B cells, and ~34% mature B cells. Bottom panel: renin-expressing cells were evaluated using the same strategy. This demonstrated that renin-expressing cells are predominantly (81.3%) pro-B cells with smaller populations of common lymphocyte progenitors (4.77%), pre-B cells (10.9%), immature B cells (6.8%) and mature B cells (0.95%). Images are representative of experiments performed in triplicate. ( g ) The percentage of renin-expressing (YFP + ) cells within the bone marrow and spleen was quantitated over time using Ren1 c -YFP mice and flow cytometry. Shortly, after birth, mice had ~0.2% renin-expressing cells. However, this percentage decreased with age in both the spleen and marrow to ~0.01%. n =8 for bone marrow samples and n =5 for spleen samples. ( h ) The percentage of renin-lineage (GFP + ) cells within the bone marrow and spleen of Ren1 dcre/+ ;mT/mG mice as measured by flow cytometry. The percentage of renin-lineage cells decreases from ~20% shortly after birth to ~2% at 200 days of life in the bone marrow. n =12 for both bone marrow and spleen samples. Full size image Next, we performed methylcellulose colony assays to define the conditions that would best permit the growth and expansion of renin-lineage cells. Cells from the bone marrow of Ren1 dcre/+ ;mT/mG mice were cultured under conditions permissive of either myeloid-erythroid or B-lymphocyte growth: cells from the renin lineage (GFP + cells) had a growth advantage in B-cell media versus myeloid-erythroid media suggesting again that renin-lineage cells are mostly B cells ( Supplementary Fig. 5b–d ). We also observed GFP + GEMM colonies in the myeloid-erythroid medium suggesting that a small number of renin precursors have myeloid potential and may be responsible for the less frequent myeloproliferative disorder we observed in a small proportion of the animals. To determine the immunophenotype of renin cells within the bone marrow, we performed flow cytometry. Bone marrow cells from Ren1 c -YFP (YFP labels cells actively transcribing renin ) [14] and Ren1 dcre/+ ;mT/mG mice (GFP labels cells, which throughout their history have expressed or continue to express renin ) were obtained and stained for lineage markers of B lymphocytes, T lymphocytes and myeloid cells and analyzed by flow cytometry. These studies demonstrated that the large majority of marrow cells that either actively express renin (YFP + cells) or are descendants from the renin-producing cells (GFP + cells) express markers of B cells (B220, CD19, IgM) with reduced expression of myeloid (Gr1 and CD11b) or T-cell (CD3) markers ( Fig. 4c,d ). YFP + cells had <10% IgM expression suggesting that renin expression occurs in early B-lymphocyte progenitors, whereas GFP + cells had ~60% IgM expression reflecting the normal maturation of renin-expressing B-lineage cells within the bone marrow. In both sets of experiments, the YFP − and GFP − cells represented a normal distribution of wild-type bone marrow ( Fig. 4e ). Additional flow strategies were performed to determine the stage of development of renin-expressing and renin-lineage cells. We quantified the number of common lymphocyte progenitors (Lin − IL7Rα + ), Pro-B cells (B220 + CD43 + ), Pre-B cells (B220 + IgM − IgD − ), Immature B-cells (B220 + IgM + IgD − ), and Mature B-cells (B220 + IgM + IgD + ) in both Ren1 c -YFP and Ren1 dcre/+ ;mT/mG mice ( Fig. 4f ). Further, we investigated the classically defined B-cell developmental subsets in the bone marrow (Hardy fractions A-F) [15] and found that renin is expressed mostly by Fraction B cells ( Supplementary Fig. 6 ). Collectively, these studies demonstrated that cells that are actively expressing renin are Pro-B cells, while renin-lineage cells, as expected, encompass premature, immature and mature B cells ( Fig. 4f and Supplementary Table 1 ). Given that RBP-J deletion occurs in B cells that currently express or previously expressed renin (provisionally, we denominated this cell as ‘B renin -cell’), we determined the relative contribution of renin-expressing cells to the cell endowment of the bone marrow and spleen at different developmental stages. We sorted cells currently expressing renin (YFP + ) and cells from the renin-lineage (GFP + ) isolated from the bone marrow and spleen of Ren1 c -YFP and Ren1 dcre/+ ;mT/mG mice described above. The fraction of renin-expressing and renin-lineage cells decreases with age both in the bone marrow and spleen ( Fig. 4g,h ). Thus, renin cells constitute a distinct subset of the total B-lymphocyte population, and their numbers diminish with age. Given the high percentage of renin-lineage cells in the spleen (~25% shortly after birth), we performed multiple experiments to further characterize the identity and stage of maturation of these cells. First, we collected spleens of Ren1 dcre/+ ;mT/mG reporter mice, stained sections with IgM antibody and evaluated by immunofluorescence. These studies demonstrated that GFP + cells in the spleen (renin-lineage) are predominantly located in the follicles, and that they represent both marginal zone (IgM bright) and follicular (IgM dim) B cells ( Fig. 5a ). Further, splenic B cells from Ren1 dcre/+ ;mT/mG mice were analysed by flow cytometry for expression of B220, CD21 and CD23. We found that GFP + cells in the spleen include both marginal zone (B220 + /CD21 Hi /CD23 Lo ) and follicular (B220 + /CD21 Int /CD23 Hi ) B cells ( Fig. 5b ), and further confirmed by staining with B220, IgM and IgD that GFP + cells mark both marginal zone (IgM Hi /IgD Lo ) and follicular (IgM Lo /IgD Hi ) B cells ( Fig. 5c ). 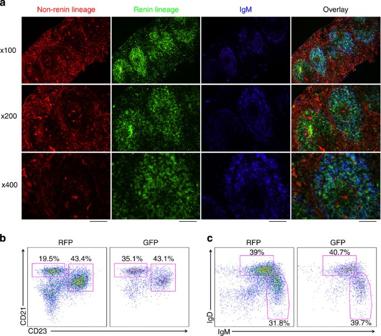Figure 5: Renin cells in the spleen represent both marginal zone and follicular B cells. (a) Fluorescence images of spleens fromRen1dcre/+;mT/mGmice. GFP+cells (renin-lineage) localize to the follicles of the spleen and largely co-localize with IgM. Scale bar, 200 μm (top row), 100 μm (middle row) and 50 μm (bottom row). (b) Flow cytometry on splenocytes fromRen1dcre/+;mT/mGmice demonstrating that renin-lineage cells (GFP+) express cell surface antigens consistent with both marginal zone (CD21HiCD23−) and follicular (CD21IntCD23+) B cells (gates are on B220+ cells). (c) Flow cytometry on spleen cells fromRen1dcre/+;mT/mGmice confirming that renin-lineage cells (GFP+) express cell surface antigens consistent with both marginal zone (IgMHiIgDLo) and follicular (IgMLoIgDHi) B cells (gates are on B220+ cells). Figure 5: Renin cells in the spleen represent both marginal zone and follicular B cells. ( a ) Fluorescence images of spleens from Ren1 dcre/+ ;mT/mG mice. GFP + cells (renin-lineage) localize to the follicles of the spleen and largely co-localize with IgM. Scale bar, 200 μm (top row), 100 μm (middle row) and 50 μm (bottom row). ( b ) Flow cytometry on splenocytes from Ren1 dcre/+ ;mT/mG mice demonstrating that renin-lineage cells (GFP + ) express cell surface antigens consistent with both marginal zone (CD21 Hi CD23 − ) and follicular (CD21 Int CD23 + ) B cells (gates are on B220+ cells). ( c ) Flow cytometry on spleen cells from Ren1 dcre/+ ;mT/mG mice confirming that renin-lineage cells (GFP + ) express cell surface antigens consistent with both marginal zone (IgM Hi IgD Lo ) and follicular (IgM Lo IgD Hi ) B cells (gates are on B220+ cells). Full size image Next, to define whether B renin -cells respond to a decrease in angiotensin II as the classical kidney renin cells, we treated Bac-ren-GFP mice [16] (here GFP identifies cells currently synthesizing renin) with the angiotensin-converting enzyme inhibitor captopril and observed by flow cytometry a 2.5-fold increase in the percentage of renin-expressing cells in the bone marrow ( Supplementary Fig. 7a ). Similarly, mice with deletion of the Ren1 d gene ( Ren1 dcre/cre ;mT/mG ) showed an increase in the number of circulating GFP + cells ( Supplementary Fig. 7b ), suggesting a recruitment of renin progenitors and their descendants both in the bone marrow and the circulation. Finally, we performed microarray analysis on renin-expressing cells sorted from the bone marrow isolated from Bac-ren-GFP mice. In addition to high expression of renin (53-fold enrichment when corrected for presorted cells), these cells displayed high expression of transcripts characteristic of precursor B lymphocytes including early B-cell factor ( Ebf1 , 13.9-fold), immunoglobulin lambda chain variable 1 ( Iglv1 , 13.8-fold), recombination-activating gene 1 ( Rag1 , 7.0-fold), pre-B-lymphocyte gene 3 ( Vpreb3 , 5.6-fold) and numerous other lymphocyte-specific transcripts displayed in abbreviated form in Table 1 . Thus, in agreement with the lineage tracing, colony-forming capacity and immunophenotyping, the microarray analysis indicated that normal renin-expressing cells in the bone marrow, the cells of origin for this type of lymphoid leukaemia, are B-lymphocyte progenitors. Table 1 Gene expression profile of B renin cells. Full size table RBP-J deletion in renin cells enriches a B-cell gene programme We next investigated how deletion of RBP-J in renin-lineage cells affects the molecular programmes regulating lymphopoiesis and contributes to leukaemogenesis. Given that the spleens of mice with leukaemia were enlarged over 15-fold due to massive infiltration with leukaemic cells, we performed microarray analysis on RNA isolated from whole spleens of control and leukaemic mice. In mice with B-cell leukaemia, genes involved in growth and differentiation of early lineage B cells ( Ebf1, Sox4 ), immunoglobulin gene rearrangements ( Vpreb1, Igll1, Rag1, Rag2 ) or cell division ( Myb ) were markedly upregulated ( Table 2 ), whereas genes that either control or are characteristic of T lymphocytes ( Tcf7, Tbx21, Art2b, CD4, CD7, Ccr9 ) were repressed when compared with control mice ( Table 2 ). We validated the mRNA expression levels for these genes by quantitative RT–PCR (qRT–PCR) and found that the qRT–PCR and microarray data expression profiles were highly correlated ( Fig. 6a,b ). In the mutant, the levels of Igll1, Enpep , Rag1 , Vpreb1 and Vpreb3 as measured by qRT–PCR were even more elevated (1,410-, 73-, 59-, 1,131- and 13–fold, respectively) than in the microarray array data, suggesting that the microarray detection had reached saturation for these transcripts. Further, we performed qRT–PCR from a pure population of cultured GFP + leukaemic cells and found a similar pattern of upregulation of genes marking early B-cell development including VpreB1, Igll1 and VpreB3 ( Supplementary Fig. 8 ). Table 2 Enrichment of a B-cell gene programme and epigenetic changes in leukaemic spleens. 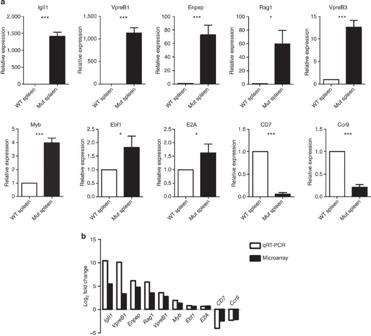Figure 6: Deletion ofRBP-Jin renin-expressing haematopoietic precursors enriches the B-cell genetic programme. (a) Validation by qRT–PCR of the differentially expressed genes in RNA from control and mutant spleens. Genes involved in early B-cell development and in T-cell and NK-cell commitment showed a remarkable difference in expression between mutant and control spleens. Error bars are s.e.m. (n=5 for each condition). Student’st-test *P<0.05; ***P<0.001. (b) Log2 values of fold changes in gene expression as measured by qRT–PCR and microarray analyses. The expression profiles were highly similar between qRT–PCR and microarray data.Igll1andVpreB1levels in the mutants are substantially higher by qRT–PCR measurements than in the array, which is likely due to the saturation of the signal in the array. Full size table Figure 6: Deletion of RBP-J in renin-expressing haematopoietic precursors enriches the B-cell genetic programme. ( a ) Validation by qRT–PCR of the differentially expressed genes in RNA from control and mutant spleens. Genes involved in early B-cell development and in T-cell and NK-cell commitment showed a remarkable difference in expression between mutant and control spleens. Error bars are s.e.m. ( n =5 for each condition). Student’s t -test * P <0.05; *** P <0.001. ( b ) Log2 values of fold changes in gene expression as measured by qRT–PCR and microarray analyses. The expression profiles were highly similar between qRT–PCR and microarray data. Igll1 and VpreB1 levels in the mutants are substantially higher by qRT–PCR measurements than in the array, which is likely due to the saturation of the signal in the array. Full size image To obtain a comprehensive view of the changes in the chromatin landscape in the leukaemic cells, we performed genome-wide ChIP-Seq analysis of chromatin from whole spleens of control and leukaemic mice using antibodies against H3K4me3 (a marker of gene activation) and H3K27me3 (a marker of gene suppression). There was remarkable congruence between this ChIP-Seq data and the mRNA array data. Table 2 shows the ratios of the average fragment density (Mutant versus Control) for H3K4me3 over the promoter from −2,500 bp to +2,500 bp relative to the transcription start and for H3K27me3 over the gene body plus 2,500 bp upstream and 5,000 bp downstream. The H3K4me3 activating marks are enriched on promoters of the upregulated genes, while there is little or no enrichment of the H3K27me3 suppressive marks. The genes downregulated in the mRNA array have diminished H3K4me3-activating marks and enrichment of H3K27me3 suppressive marks. 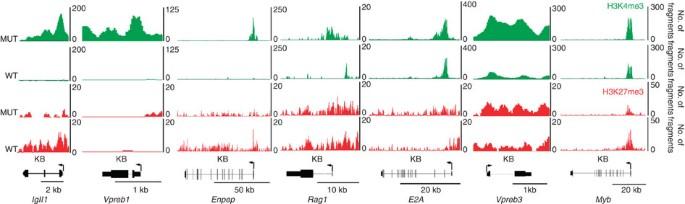Figure 7: Chromatin profiles of genes activated in the mutant leukaemic spleen. The profiles depict the ChIP-Seq signals for H3K4me3 (green) and H3K27me3 (red) modifications in mutant (MUT) and wild-type (WT) spleens. Thexaxis for all genes is in KB with the scale indicated by the bar below each gene. Theyaxis corresponds to the number of sequenced ChIP fragments that overlap a given position. The highly upregulated genes in the mutant all display increased occupancy of the H3K4me3 activation mark on the promoter and, in the case ofVpreb1, Vpreb3andIgll1, throughout the gene. In contrast, in the WT those genes have low or no occupancy of activating marks. The H3K27me3 suppressive mark is consistently lower than the activation mark in the MUT. Figure 7 shows the pattern of modifications on the upregulated genes validated previously by qRT–PCR. The highly upregulated genes in the mutant cells display increased presence of the H3K4me3 activation mark on the promoter and, in the case of Vpreb1, Vpreb3 and Igll1 , throughout the gene ( Fig. 7 ). In wild-type cells, these genes have low or no occupancy of activating marks. Further, the H3K27me3 suppressive mark is consistently lower than the activation mark in the mutant. In summary, the mRNA array, qRT–PCR and ChIP-Seq results demonstrate that genes important for commitment to early B-cell development are markedly upregulated, whereas genes associated with other haematopoietic lineages are repressed when compared with control mice. Thus, deletion of RBP-J in renin-expressing haematopoietic precursors leads to enrichment of precursor B-lineage genes at the expense of alternative cell fates, a process facilitated by epigenetic changes. Figure 7: Chromatin profiles of genes activated in the mutant leukaemic spleen. The profiles depict the ChIP-Seq signals for H3K4me3 (green) and H3K27me3 (red) modifications in mutant (MUT) and wild-type (WT) spleens. The x axis for all genes is in KB with the scale indicated by the bar below each gene. The y axis corresponds to the number of sequenced ChIP fragments that overlap a given position. The highly upregulated genes in the mutant all display increased occupancy of the H3K4me3 activation mark on the promoter and, in the case of Vpreb1, Vpreb3 and Igll1 , throughout the gene. In contrast, in the WT those genes have low or no occupancy of activating marks. The H3K27me3 suppressive mark is consistently lower than the activation mark in the MUT. Full size image Gene set enrichment analysis (GSEA) is a computational method that determines whether defined gene signatures are differentially expressed between two groups [17] . Using a canonical pathway knowledge database containing 880 known gene sets, we performed GSEA on our gene expression data comparing the expression pattern in spleens from mice with leukaemia versus control mice. Cells from mice with leukaemia were enriched in gene signatures associated with cell cycle progression ( Supplementary Fig. 9a and Supplementary Table 2 ). Flow cytometry confirmed that mutant cells have an increased percentage of cells in the S and G2/M phases compared with control cells, indicating enhanced cell division as a result of RBP-J deletion ( Supplementary Fig. 9b,c ). Further, phosphohistone H3 staining showed a higher number of cells undergoing proliferation in leukaemic versus control mice ( Supplementary Fig. 9d,e ). These results indicate that deletion of RBP-J promotes cell cycle progression and cellular proliferation in B cells. Together, these results show that silencing of RBP-J in renin-expressing cells restricts the lineage potential of these progenitors to a precursor B-cell fate and alters the regulation of cell cycle progression ultimately leading to leukaemic transformation. Mutations of RBP-J in patients with lymphoid malignancies Given the striking findings encountered in our mice, we investigated whether mutations of RBP-J are present in human haematological malignancies. We performed RBP-J exon sequencing in 44 patients with confirmed haematopoietic malignancies ( Supplementary Table 3 ). A total of 10 patients (23%) had variants in the coding region of RBP-J ( Supplementary Table 4 ). We identified nine different predicted missense mutations and two frameshift deletions ( Supplementary Fig. 10a ). One deletion recurred in five patients, causing a frameshift at position 188 of the coding region, which is predicted to result in a 104 amino-acid truncated protein. These variants occurred in highly conserved regions of RBP-J and are novel as none of them were found in a large number of normal genomes including 1000 Genomes Project, NCBI Single-Nucleotide Polymorphism database (dbSNP) and NHLBI Exome Sequencing Project (ESP5400). Finally, many of the missense variants are predicted to be damaging to the protein product as determined by multiple prediction models including AVSIFT, SIFT, PolyPhen2, LRT and Mutation Taster ( Supplementary Table 4 ). Of note, RBP-J variants occurred in both B-cell and myeloid malignancies ( Supplementary Fig. 10b ). Mice with deletion of RBP-J in renin cells develop precursor B-cell leukaemia. The cell of origin for this leukaemia is a novel renin-expressing haematopoietic progenitor with a B-lymphocyte pedigree, which we have termed the B renin -cell. Deletion of RBP-J in these precursors leads to enrichment of the genetic programme for B-cell commitment, enhanced cell cycle progression and proliferation, infiltration of multiple organs and early death. Leukaemic cells have clonal IgH rearrangements, can be cultured for multiple passages, are transplantable in irradiated animals and can be recovered from recipient mice and further grown in culture. To our knowledge, this is the first report demonstrating RBP-J silencing as an initiating event in B-cell leukaemogenesis. Radke et al. [18] showed that deletion of Notch1 in adult bone marrow results in enhanced B-cell development, but not overt leukaemia. Han et al. [11] used Mx-Cre mice to delete RBP-J in adult bone marrow cells resulting in blockade of T-cell development and increase in B-cell development within the thymus, but not leukaemia. Finally, Tanigaki et al. [19] deleted RBP-J in B-cells by targeting the B-cell lineage marker CD19, leading to enhanced follicular B-cell populations with loss of marginal zone B-cells but no leukaemia phenotype. Remarkably, deletion of RBP-J in B renin -cells leads to overt leukaemia suggesting that these renin-expressing cells are particularly vulnerable to transformation. However, we have not excluded the possibility that the precursor B leukaemia observed in the current study reflects strain differences in our mice compared with other conditional models of RBP-J deletion that do not result in leukaemia. The existence of a local bone marrow renin-angiotensin system (RAS) has previously been described [20] . Components of the RAS are present in bone marrow cells with putative roles in both normal and neoplastic haematopoiesis [21] , [22] , [23] , [24] . While the presence of renin in the bone marrow has been suggested, the identity and function of renin cells during haematopoiesis were unknown. In our study, we found that B renin -cells decrease from ~20 to ~1% in the normal bone marrow and from ~20 to ~5% in the spleen by 6 months of age. Further, a related member of the RAS, angiotensin-converting enzyme (ACE), has been well characterized as a marker of haematopoietic stem cells during both fetal and adult life [25] , [26] . It is therefore possible that B renin -cells may be remnants of embryonic haematopoiesis or that renin marks a specific stem cell population with differential transforming capacity, accounting for the difference between models [27] , and suggesting that the phenotype caused by loss of RBP-J in haematopoietic cells depends on the cell of origin. Together with previous studies, our findings suggest that renin and the RAS may play critical roles in haematopoietic ontogeny and HSC plasticity. We found remarkable developmental, biochemical/ transcriptional and functional similarities between the B renin -cell and its seemingly more distant kidney renin cell. Similar to their kidney cell counterpart, B renin -cells in the bone marrow and spleen also decrease in number as development proceeds and are responsive to physiological challenges: captopril treatment as well as life-time deletion of the Ren1 d gene disturbs circulatory and fluid-electrolyte homeostasis and induce an increase in GFP + cells in the bone marrow and the circulation indicating that renin-expressing haematopoietic cells respond to systemic and/or local physiological cues, such as lack of angiotensin, in a manner not dissimilar to the JG cell [6] . B renin -cells and JG renin cells also share numerous transcriptional regulators, notably EBF1 , a known regulator of lymphocyte development, members of the Notch pathway including ligands and receptors and the final transcriptional effector, RBP-J [14] . These observations suggest conservation of the regulatory machinery and a possible lineage relationship between the two cell types. The functional relevance of these findings is underscored by the fact that both cell types need RBP-J to differentiate and function properly: lack of RBP-J in kidney renin cells results in a significant decrease in the number of renin cells and loss of the descendant’s memory to regain the renin phenotype. Similarly, mutant B renin -cells lose their differentiation potential, are retained in a precursor stage and lose control of their normal cell cycle leading to neoplastic transformation. In both cases, RBP-J regulates cell fate. What is the local function of renin precursors in these two tissues? In the kidney, renin cells control vascular development [28] , [29] , [30] , [31] . Although components of the renin–angiotensin system have been described in peripheral leukocytes [22] and bone marrow [23] , the function of renin cells in haematopoietic tissues remains to be determined. It would be interesting to determine whether B renin cells also participate in the coordinated systemic response to control circulatory and fluid-electrolyte homeostasis, or whether renin expression in the bone marrow serves some other role during primitive, definitive and neoplastic haematopoiesis [23] . In this study, we found cooperative mechanisms for leukaemic transformation: upregulation of genes involved in B-cell specification and of genes involved in cell cycle progression. During normal haematopoiesis, Notch/RBP-J signalling favours T-cell development by repressing a network of transcription factors important for early B-cell commitment including EBF1 and E2A [27] , [32] , [33] , [34] . These transcription factors in turn are responsible for activating transcription of several genes critical for early B-cell development, including Igll1 , Rag1 and Vpreb1 (ref. 35 ). Deletion of RBP-J in renin cells led to increased expression of those B-lineage associated transcripts. These findings were correlated with ChIP-Seq data. H3K4me3 activating marks, which facilitate the opening of the chromatin structure to permit transcription, were present along those genes responsible for the pre B-cell genetic programme. Of note are the highly overexpressed genes Rag1 , Vpreb1 and Vpreb3 that had H3K4 activation marks not only in the promoter but also along the entire body of gene reinforcing their open chromatin structure. In addition, the ChIP-Seq data showed H3K27 repressive marks along genes from other lineages. Thus de-repression of the determinants of B-lineage commitment by deletion of RBP-J appears to restrict progenitors to a precursor B-cell fate. Our array and GSEA analyses also demonstrated enrichment of genes involved in cell cycle progression. Genetic defects that cause a block in lymphocyte differentiation and progression of the G1/S cell cycle transition have been reported in lymphocytic leukaemia [36] , [37] . Similar to these findings, deletion of RBP-J in B renin -cells leads to cell cycle progression and increased cellular proliferation, tissue infiltration and early death. Mutations of RBP-J in humans have not been extensively studied: we could find only one report of an RBP-J sequence mutation occurring in a haematologic malignancy [38] . Schuh et al. [38] performed whole-genome sequencing to track the subclonal evolution of chronic lymphocytic leukaemia in three patients over different treatment time points. They identified a mutation occurring in RBP-J in a single patient, and, similar to our findings, this variant was present at a low frequency (1.16 to 6.69% over different time points). To further explore whether mutations in RBP-J contribute to human disease, we sequenced the exome of RBP-J in 44 bone marrow specimens from patients with haematopoietic malignancies. We found that a fraction of B-cell malignancies contained single-nucleotide variants in the coding regions of RBP-J . These variants occurred in conserved regions of the gene, have not previously been seen in a large number of healthy individuals and are predicted to have negative translational consequences. In addition, we detected RBP-J variants in myeloid leukaemia samples that support previous work demonstrating inactivating mutations of the Notch pathway in patients with chronic myelomonocytic leukaemia [39] . Several limitations of this study are worth noting. First, we did not have remission samples from these patients to confirm the somatic nature of these mutations. Second, the bone marrow samples likely included a mixed population of cells including normal haematopoietic cells and heterogeneous malignant subclones, which may have influenced the low variant allele frequency. However, the significant occurrence of these RBP-J variants in a variety of haematologic malignancies in this and the aforementioned study [38] and the fact that these variants have not been previously detected in healthy individuals suggest that mutations of RBP-J should be further studied to define whether they indeed contribute to disease development, maintenance or progression in humans. In summary, we identified novel bone marrow progenitors, which express renin and become the source of lymphoblastic leukaemia when RBP-J is missing ( Fig. 8 ). The possibility that within the B-cell population there are subsets of progenitors with differential transformative capacity has significant implications for understanding the origin of leukaemia. The discovery of these progenitors, the reproducibility of this highly penetrant mouse model of leukaemia, and the generation of a new GFP labelled leukaemia cell line offer an invaluable opportunity to explore the mechanisms responsible for normal and neoplastic haematopoiesis. 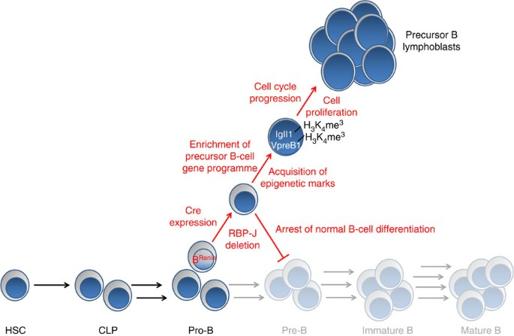Figure 8: Depiction of this model of lymphoblastic leukaemia. Normal B-cell development proceeds from haematopoietic stem cells (HSC) through multiple stages to ultimately become mature B cells. A small subset of pro-B cells express renin and are termed BRenin-cells. In this model, activation of the renin promoter in BRenin-cells results incre recombinaseexpression and subsequentlyRBP-Jdeletion. These cells fail to differentiate along the normal B-cell pathway, undergo epigenetic activation and enrichment of a precursor B-cell gene programme. Mutant cells additionally experience cell cycle progression and cell proliferation ultimately resulting in expansion of a lymphoblast population and the development of precursor B cell leukaemia. Figure 8: Depiction of this model of lymphoblastic leukaemia. Normal B-cell development proceeds from haematopoietic stem cells (HSC) through multiple stages to ultimately become mature B cells. A small subset of pro-B cells express renin and are termed B Renin -cells. In this model, activation of the renin promoter in B Renin -cells results in cre recombinase expression and subsequently RBP-J deletion. These cells fail to differentiate along the normal B-cell pathway, undergo epigenetic activation and enrichment of a precursor B-cell gene programme. Mutant cells additionally experience cell cycle progression and cell proliferation ultimately resulting in expansion of a lymphoblast population and the development of precursor B cell leukaemia. Full size image Generation of study mice To inactivate RBP-J in renin-lineage cells, we crossed Ren1 dcre/+ mice [1] , which express Cre recombinase in renin cells, to RBP-J floxed ( RBP-J fl/fl ) mice (a kind gift from T Honjo) [11] . Mice carrying both RBP-J fl/fl and Ren1 dcre/+ undergo Cre -mediated recombination specifically in cells that express renin leading to deletion of RBP-J [11] , [19] . RBP-J fl/+ ;Ren1 dcre/+ mice were mated to generate RBP-J fl/fl ;Ren1 d+/+ (control) and RBP-J fl/fl ;Ren1 dcre/+ (mutant) mice. For genotyping, genomic DNA was extracted and purified from tail biopsies using Quiagen DNeasy Blood and Tissue kit (Valencia, CA) according to the manufacturer’s instructions, and standard PCR was performed in an Eppendorf thermocycler using Taq polymerase (Promega, Madison, WI). The primers used for genotyping were: wild-type renin forward 5′-GAAGGAGAG CAAAAGGTAAGAG-3′, wild-type renin reverse 5′-GTAGTAGAAGGGGGAGTTGTG-3′, Ren1 dcre forward 5′-GAAGGAGAGCAAAAGGTAAGAG-3′, Ren1 dcre reverse 5′-TTGGTGTACGGTCAGTAAATTGGAC-3′, wild-type RBP-J forward 5′-GTTCTTAACCTGTTGGTCGGAACC-3′, wild-type RBP-J reverse 5′-GCTTGAGGCTTGATGTTCTGTAATGC-3′, floxed RBP-J forward 5′-GTTCTTAACCTGTTGGTCGGAACC-3′, and floxed RBP-J reverse 5′-GCAATCCATCTTGTTCAATGGCC-3′ (ref. 10 ). Lineage tracing was performed to determine the pattern of renin expression in the bone marrow and spleen. Ren1 dcre/+ mice were bred to the lineage reporter line mT/mG [12] . In this reporter, non-recombined cells express RFP, and following Cre- mediated recombination GFP is expressed in renin-lineage cells and their descendants. This line was used to isolate renin-lineage cells in normal mice and in mice with RBP-J deletion within renin cells. Ren1 c -YFP transgenic mice were used to isolate cells that actively express renin [40] . Finally, renin-expressing cells in the bone marrow were isolated for gene array studies from transgenic Bac-Ren1 c -GFP mice [16] . Flow cytometry and immunofluorescence experiments involving renin-expressing and renin-lineage reporters were performed on both male and female mice between the age of 2 weeks and 3 months. To determine the relative fraction of renin cells within the bone marrow and spleen at different developmental stages, renin-expressing and renin-lineage mice were evaluated at different ages between 2 weeks and 200 days of life. Mutant mice were monitored until they developed signs and symptoms of disease. When they became moribund, they were anaesthetized with tribromoethanol (300 mg kg −1 ) [41] , and organs were removed, preserved for RNA extraction, fixed for immunohistochemistry or immunofluorescence, or processed for flow cytometry. Twenty-four mutant mice are included in this study with equal numbers of age-matched control animals. Study animals included both males and females. All procedures were performed in accordance with the National Institutes of Health guidelines for the care and use of laboratory animals and were approved by The Animal Care and Use Committee of the University of Virginia. Identification of cell phenotypes by flow cytometry To determine the subtype of leukaemia and characterize its cell of origin, flow cytometry analysis was performed. Single-cell suspensions were obtained from the bone marrow, spleen and tumours found in the abdomen and axillary regions. To obtain bone marrow cells, the long bones of mice were dissected, flushed with cell suspension media (Biolegends, San Diego, CA), and the cells were passed through a 70 μm strainer. Spleens or tumours were dissected cleanly, placed on a 70 μm strainer and, using the plunger end of a syringe, gently passed through the strainer. The tissue was rinsed with cell staining buffer (CSB) (Biolegends) and the process repeated until the spleen capsule turned clear. All cells were treated with RBC lysis buffer (Sigma, St Louis, MO), resuspended in CSB, counted using a haemocytometer and distributed into microcentrifuge tubes for antibody labelling against the surface markers in Supplementary Table 5 (all antibodies were purchased from Biolegends except CD43, which was purchased from Becton Dickinson, Franklin Lakes, NJ). Antibodies were added at predetermined optimum concentrations ( Supplementary Table 5 ) and incubated at room temperature for 20 min. Immunophenotyping was performed in the UVA Flow Cytometry core lab using a Fortessa cytometer and data analysed with FlowJo program. Identification of RBP-J deletion in peripheral blood To mark with GFP and indirectly evaluate the deletion of RBP-J in circulating leukocytes, 0.5 μl of blood from RBP-J fl/fl ;Ren1 dcre/+ ;mT/mG and RBP-J +/+ ;Ren1 dcre/+ ;mT/mG mice was obtained by a small cut of the tip of the tail, collected using heparinized pipette tips and diluted in 100 μl of cold PBS in a 96-well plate. Using an inverted microscope (Leica DMIRE2) recombined (GFP + ) and not recombined (RFP + ) cells were counted in three fields using a × 20 objective and pictures were taken using a Retiga EXi camera (Q-Imaging, Surry, BC). RNA extraction and PCR analysis Total RNA was isolated from the whole bone marrow, spleen and tumour samples using Trizol extraction (Life Technologies, Grand Island, NY) according to the manufacturer’s instructions. cDNA was prepared from 2 μg of RNA using Moloney murine leukaemia virus reverse transcriptase (Life Technologies, Grand Island, NY) and an oligo(dT) primer according to the manufacturer’s instructions. PCR was performed on 2 μl of cDNA using Taq DNA polymerase (Promega, Madison, WI) [40] . For validation of microarray data, qPCR was performed using SYBR Green 1 (Invitrogen Molecular Probes, Eugene, OR) in a CFXConnect system (Biorad, Hercules, CA) [42] . Primers are listed in Supplementary Table 6 . Histologic analysis Immunohistochemistry was performed on Bouin’s and formalin-fixed tissue. In brief, 5-μm tissue sections were deparaffinized in xylenes and graded alcohols. Sections were incubated overnight with primary antibodies against PAX5 (BD Clone 24/Pax5, dilution 1:40), CD79a (Dako Clone JCB117, dilution 1:400), TdT (Cell Marque polyclonal, ready to use), CD34 (Dako Clone QBEnd10, dilution 1:100) and Phosphohistone H3 (Cell Signaling Technologies, dilution 1:200), and antibody binding was visualized using the Vectastain ABC kit (Vector Laboratories, Burlingame, CA). Sections were counter-stained with haematoxylin, dehydrated through graded alcohols to xylenes and mounted with Permount. Immunofluorescence was performed on frozen sections using a primary antibody against IgM (Biolegends, dilution 1:10). Sections were washed with PBS then blocked for 1 h using 10% BSA in PBS with 1% normal donkey serum. The primary antibody was incubated overnight at 4 °C then incubated with a fluorescently conjugated secondary antibody (AlexaFluor 350, Invitrogen, 1:500). Immunoglobulin gene rearrangement analysis Genomic DNA from the bone marrow, spleen and tumour samples was used as templates for PCR amplification. Primer pairs used were DQ52 for 5′-CCACAGGCTCGAGAACTTTAGCG-3′; J H 4 Rev 5′-AGGCTCTGAGATCCCTAGACAG-3′ to detect D-J recombination products; V H 7183 for 5′-GTGGAGTCTGGGGGAGGCTTA-3′; J H 4 Rev 5′-AGGCTCTGAGATCCCTAGACAG-3′ to detect V-DJ products; DLG5 for 5′-AAGTCTCAGGCTGGCCATTA-3′; DLG5 Rev 5′-TTTACCACCCCTGACACACA-3′ to amplify a single-copy gene used for normalization of DNA amount [43] . The PCR reaction was performed in a 50 μl volume containing 100 ng, 33 ng or 11 ng of template DNA, 1 × PCR buffer, 1.5 mM MgCl 2 , 0.2 mM dNTPs, 0.4 μmM each primer and 0.75 U Taq polymerase (Promega Corporation, Madison, WI). Thermocycling conditions were as follows: 4 min at 95 °C followed by 31 cycles of 30 s at 95 °C, 90 s at 60 °C, 2 min at 72 °C and a final extension step of 5 min at 72 °C. Products (15 or 20 μl of the PCR reaction) were separated on 1% agarose gels, transferred to GeneScreen Plus Hybridization Transfer Membrane (Perkin Elmer, Waltham, MA) and hybridized at 42 °C to J H probe 5′-TATGGACTACTGGGGTCAAGGAA-3′end labelled with 32 P-ATP using 20 U of T4 polynucleotide kinase (New England Biolabs, Ipswich, MA). Membranes were washed with 2 × SSC, 0.1% SDS and exposed to Kodak Biomax MS film. Cell cycle analysis The DNA content of fixed cells from the bone marrow and spleen was determined using propidium iodide (PI) staining [44] . Single-cell suspensions from the spleen and bone marrow were obtained as described above. The cells were counted using a haemocytometer, and 1 × 10 6 cells were fixed and stored in 70% ethanol at 4 °C. On the day of cell cycle analysis, the fixed cells were resuspended in 5 ml PBS, centrifuged 5 min at 200 × g and resuspended in 1 ml of PI staining solution (10 ml of TritonX-100 PBS, 2 mg DNase-free RNase A and 200 μl of 1 mg ml −1 PI). Cells were incubated in PI solution for 30 min at room temperature, and DNA content was determined using flow cytometry. In vitro colony-forming assay To determine the growth characteristics of renin-lineage cells, bone marrow cells from Ren1 dcre/+ ;mT/mG reporter mice were grown in methylcellulose with medium permissive for either B-lymphocyte or myeloid-erythroid colony growth (Methocult GF medium for mouse Pre-B cells, M3630, and Methocult GF for mouse haematopoietic progenitors, M3434, StemCell Technologies Vancouver, BC, Canada). Cells were diluted in Iscove’s MDM with 5% FBS, and plated in duplicate samples at 1 × 10 5 cells per 30 mm plate. After incubation for 14 days at 37 °C in 5% humidified CO 2 , plates were visualized using inverted microscopy (Leica DMIRE2) and colony-forming units (CFUs) were scored according to standard criteria [45] . The percent of GFP + (renin-lineage) colonies was quantitated in both B-cell and myeloid/erythroid permissive culture conditions. Transplantation studies Leukaemic B cells that express GFP were purified from methylcellulose cultures and injected intravenously at a dose of 2–6 × 10 6 cells into irradiated mice (13 Gy) ( n =3). Recipients were monitored closely and killed at 1 week post injection. Control animals included non-irradiated mice that received leukaemic cell injections, and irradiated mice that received vehicle only (media). Gene expression analysis RNA was isolated from spleens from mutant and control mice. Hybridization to the Affymetrix mouse gene array ST1.0 was performed by the UVA Core Lab Microarray Facility. All preprocessing and analysis were done using R version 2.15.0. CEL files were imported using the Affymetrix package, version 1.34.0. Expression intensities were summarized, normalized and transformed using Robust Multiarray Average algorithm [46] . Probesets were annotated using the BioConductor annotation package mogene10sttranscriptcluster.db version 8.0.1, annotate package, version 1.34.0. Linear models with empirical Bayes moderated standard errors were fit using the BioConductor limma package version 3.12.1. False discovery rate was used to correct for multiple testing. Gene set enrichment analysis was used to examine coordinated gene expression changes in canonical pathways using the Molecular Signatures Database curated canonical pathway gene set [17] , [47] . GEO accession: GSE46229 . RNA was extracted from renin-expressing bone marrow cells isolated from Bac-Ren1 c -GFP mice using a Becton-Dickinson Aria 2 cell sorter in the RPCI Flow Cytometry Core Facility. RNA from unsorted bone marrow and GFP + cells was hybridized to MOE430 V2.0 oligonucleotide microarray GeneChip Arrays (Affymetrix) in the RPCI Gene Expression Facility. The results from the three replicates were normalized using RMA and quantile. GEO accession: GSE53916 . Chromatin immunoprecipitation and next generation sequencing Chromatin immunoprecipitation (ChIP-Seq) was performed by Active Motif (Carlsbad, CA). Chromatin (30 μg) from control and mutant spleens was precipitated with antibodies against H3K4me3, a marker of active genes (2 μl, AM 39159) and H3K27me3, a marker of inactive genes (4 μl, Millipore 17–449). ChIP DNA was processed into Illumina libraries using standard procedures, and libraries were sequenced on HiSeq 2000. The 50-nt sequence reads were mapped to the mouse mm9 genome using the BWA algorithm with default settings. For the analysis, all data files were normalized to the same number of unique alignments without duplicate reads (17.5 million). Sequence tags were extended in silico (using Active Motif software) at their 3′-ends to a length of 200 bp. To identify the density of fragments (extended tags) along the genome, the genome was divided into 32-nt bins and the number of fragments in each bin was determined. The resulting histogram files were used to extract average fragment density values for predefined promoter and gene regions. For H3K4me3, promoter regions from −2,500 bp to +2,500 bp relative to the transcription start sites were used. However, for Vpreb1, the promoter regions were restricted to −500 bp to +500 bp relative to the transcription start site to discriminate Vpreb1 from the nearby gene, Top3b . For H3K27me3, gene regions plus 2,500 bp upstream and 5,000 bp downstream flanking regions were used. In this approach, the same genomic segments are compared between the Mutant and Control data sets, and the ratio of average fragment densities is a valid metric for comparison. In parallel, genomic regions with significant enrichments in tag numbers were identified using the SICER peak finding algorithm49 (cutoff FDR, 1E-10). Only genes with SICER peaks were included in the ratio calculation described above and shown in the Table 2 . GEO accession: GSE46566 . RBP-J Sequencing in Human Bone Marrow Specimens To identify mutations in RBP-J that may be causing loss of function in human disease, we performed RBP-J exon sequencing in the bone marrow from patients with haematopoietic malignancies. Genomic DNA was isolated from 140 bone marrow samples using the Qiagen DNAeasy kit, and 84 samples were suitable for sequencing. Amplicons were designed Using TruSeq Custom Amplicon design studio to cover the coding regions of RBP-J and exome enrichment was performed. After PCR amplification, each exon was sequenced using an Illumina MiSeq instrument with paired-end 151 base pair reads. Data were aligned using MiSeq Reporter version E. All variants that were non-synonymous were evaluated for significance. Of these 84 samples, 44 patients had a definitive diagnosis of haematopoietic malignancy available in their medical record and were included in our analysis. These studies were approved by the University of Virginia Institutional Review Board for Health Science Research. The project met criteria of research involving coded biological specimens, and informed consent was not required. Statistical analysis Data are presented as means±s.e.m. Significance between groups was determined using the Mann–Whitney U -test and two-tailed Student’s t -test using GraphPad Prism 5.0. Differences were considered statistically significant at the * P <0.05; ** P <0.01 and *** P <0.001 levels. Accession codes: Microarray expression data have been deposited in the Gene Expression Omnibus database under accession: codes GSE46229 and GSE53916 . The CHiP-seq data have been deposited in the Gene Expression Omnibus database under accession: code GSE46566 . How to cite this article: Belyea, B. C. et al. Identification of renin progenitors in the mouse bone marrow that give rise to B-cell leukaemia. Nat. Commun. 5:3273 doi: 10.1038/ncomms4273 (2014).